3D optical Yagi–Uda nanoantenna array Future photonic circuits with the capability of high-speed data processing at optical frequencies will rely on the implementation of efficient emitters and detectors on the nanoscale. Towards this goal, bridging the size mismatch between optical radiation and subwavelength emitters or detectors by optical nanoantennas is a subject of current research in the field of plasmonics. Here we introduce an array of three-dimensional optical Yagi–Uda antennas, fabricated using top-down fabrication techniques combined with layer-by-layer processing. We show that the concepts of radiofrequency antenna arrays can be applied to the optical regime proving superior directional properties compared with a single planar optical antenna, particularly for emission and reception into the third dimension. Measuring the optical properties of the structure reveals that impinging light on the array is efficiently absorbed on the subwavelength scale because of the high directivity. Moreover, we show in simulations that combining the array with suitable feeding circuits gives rise to the prospect of beam steering at optical wavelengths. Nanoantennas are links between an emitter or detector and free-space propagation of light. Such nanostructures have gained considerable attention over the past few years by scaling down well-established concepts of the high-frequency electromagnetic spectral region into the nanoscale optical region [1] , [2] , [3] , [4] , [5] . Designs including nanorods [6] , [7] , bow-tie antennas [8] , patch antennas [9] or planar Yagi–Uda antennas [10] , [11] , [12] , [13] have been recently demonstrated. Antennas in the radio- and microwave region are widely used to tailor the emission pattern of electromagnetic sources and also, by reciprocity, to collect radiation efficiently from defined directions [14] , [15] . Metallic nanoparticles with their plasmon resonances in the optical wavelength region can be used in a similar manner. Near-field coupling of quantum emitters to these particle plasmon resonances is used to redirect the light emission, and the far-field radiation is completely determined by the antenna mode [16] , [17] . The redirection of emission is quantified by the expression of directivity [14] which is the power P ( θ,φ ) per unit solid angle emitted in a given direction divided by the emitted power per solid angle by an isotropic source of equal total radiated power. A promising antenna geometry for tailoring the emission pattern is the Yagi–Uda antenna, which is widely used in GHz communication because of its high maximal directivity [18] . Recent theoretical and experimental studies have shown that the concept of the Yagi–Uda antenna can be applied to optical frequencies [19] , [20] and the emission of dipole emitters on the nanoscale can be redirected [10] , [12] , [13] , [17] . In these studies, the authors investigate single optical Yagi–Uda antennas in which they use nanorods, nanodisks, core-shell particles and nanospheres as building elements of the antenna. Here we demonstrate theoretically and experimentally a three-dimensional (3D) stacked Yagi–Uda antenna array, which can direct optical emission into the third dimension. We fabricate a large-area array of such nanoantennas and simulate its directivity properties, exceeding largely the values of just the single Yagi–Uda antenna. Measuring experimentally the optical spectra of the antenna array reveals the directive absorption of light in the feed elements of the Yagi–Uda antennas in the array. We compare the measurements with theory and propose to use such nanoantenna arrays as optical phased array emitters or receivers [14] , which would find useful applications in direct optical links of future nanophotonic circuits. 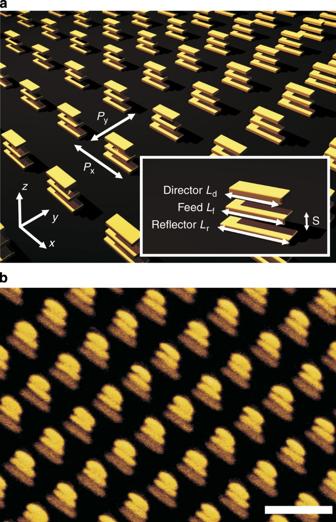Figure 1: The optical Yagi–Uda antenna array. (a) Schematic picture of the optical Yagi–Uda antenna array. The period inx-direction isPx=450 nm and iny-directionPy=300 nm. The inset shows the single antenna with definitions of the geometrical parameters:Lr=300 nm,Lf=250 nm,Ld=230 nm andS=100 nm. (b) Scanning electron microscope image of the optical Yagi–Uda antenna array. The gold structure is fabricated on a glass substrate. The nanorods are embedded in a photopolymer (PC403), which serves as the dielectric spacer. Scale bar, 500 nm. Top-down fabrication of the 3D antenna structure Figure 1a shows a schematic picture of the array, in which the period is chosen to be 450 nm in x -direction and 300 nm in y -direction. The inset depicts the geometry of the single three-layer Yagi–Uda antenna in the array, in which the central element is the feed ( L f =250 nm) sandwiched between the back reflector ( L r =300 nm) and the front director ( L d =230 nm). The distance between each layer is 100 nm. Figure 1: The optical Yagi–Uda antenna array. ( a ) Schematic picture of the optical Yagi–Uda antenna array. The period in x -direction is P x =450 nm and in y -direction P y =300 nm. The inset shows the single antenna with definitions of the geometrical parameters: L r =300 nm, L f =250 nm, L d =230 nm and S =100 nm. ( b ) Scanning electron microscope image of the optical Yagi–Uda antenna array. The gold structure is fabricated on a glass substrate. The nanorods are embedded in a photopolymer (PC403), which serves as the dielectric spacer. Scale bar, 500 nm. Full size image The antenna array (size 90×90 μm), shown in the scanning electron microscope picture of Figure 1b , is fabricated with electron beam lithography (EBL) on a glass substrate, using the layer-by-layer stacking method introduced by Liu et al . [21] At least three gold alignment marks (size 4×80 μm) with a gold thickness of 250 nm are first fabricated on a quartz substrate. Next, nanorod structures are defined in positive resist (polymethyl methacrylate, PMMA) by electron-beam lithography. After evaporation of a 30-nm gold film and subsequent lift-off, a 100-nm-thick spacer layer is applied on the first layer by spin coating. For this step we use a solidifiable photo polymer PC403 (JCR) as the planarizing spacer layer. A pre-baking process by continuously increasing the baking temperature from 90 to 130 °C is first performed to remove the solvent from the polymer. A sufficiently long bake at a higher temperature (60 min in a 180 °C oven) further hardens the layer. PMMA is subsequently spin coated onto the sample and the stacking alignment using the gold alignment marks is applied to ensure the accurate stacking of the second nanorod layer. Subsequently, the procedures of planarization and in-plane fabrication are repeated for the third layer. With a final layer of PC403, we produce a completely embedded structure. Recently, it was shown experimentally that one single-optical Yagi–Uda antenna achieves a narrow emission along its antenna axis in the substrate plane [19] or into the critical angle of the substrate, with a strong preference towards the antenna axis [20] . By stacking of the Yagi–Uda elements, we are able to direct the antenna axis and thus the emission out of the substrate plane ( z -direction). It also provides us the opportunity to array several Yagi–Uda antennas in the other two dimensions, which renders our structure truly 3D. Similar to the radiowave and microwave region, in which antenna arrays are often used to increase the directivity, we expect to sharpen the radiation pattern in two directions compared with the emission of the single antenna. Numerical calculations of redirected emission cone The angular pattern of the whole array is the product of the angular element pattern and the array factor, which is the angular radiation pattern of isotropic point sources with the same spatial distribution as the antennas in the array [14] . 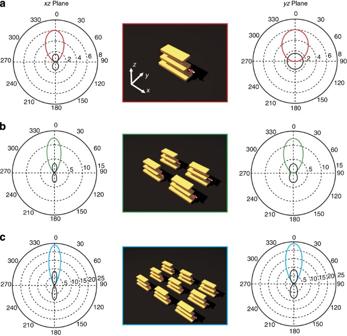Figure 2: Numerical directivity of the transmitting Yagi–Uda array coupled to dipole emitters. The polar plots show the numerically calculated directivity for (a) a single optical Yagi–Uda antenna, (b) a 2×2 array and (c) a 3×3 array. The calculated directivity of thexzplane is plotted in the left column and for theyzplane in the right column. Each antenna is fed by a dipole source (red spheres, 5 nm away from the feed element) with a dipole moment along thex-direction. The emitted wavelength of the dipole is 1500 nm. The black curves in the polar plots are the directivities of the corresponding emitter array without being coupled to optical antennas. Nevertheless, in the simulations shown in Figure 2 , we implement the complete array configuration into the calculation domain to account for mutual coupling effects between the Yagi–Uda antennas in the array, which are not accounted for by simple pattern multiplication. Each feed element is coupled to a dipole emitter (red sphere in Fig. 2 ) at a distance of 5 nm from the nanorod, emitting at λ =1.5 μm and oscillating in the direction of the nanorod axis indicated by the white rod in the schematic view. The antennas are embedded in a dielectric environment with refractive index n =1.55, taking into account the dielectric spacer used in the fabrication. In the left column of Figure 2, the directivity pattern in the xz plane is plotted, whereas the right column shows the directivity pattern in the yz plane. Figure 2a is the single Yagi–Uda antenna case. The red curve is the directivity of the antenna coupled to the dipole emitter and the black curve shows the directivity pattern of the single dipole emitter without the antenna. To obtain maximum radiation at λ =1.5 μm into the z -direction, we vary the geometrical parameters of the single Yagi–Uda antenna. First, we consider just the feed element coupled to the dipole emitter ( λ =1.5 μm) and maximize the radiated power by changing the length of the gold nanorod. The coupling between dipole emitter and nanorod is strongest for a rod length of 250 nm and the symmetric far-field radiation is completely determined by the dipole mode of the feed element. As a second element, a slightly longer gold rod, the reflector, is placed underneath the feed element. As the structure symmetry is now broken along the z -axis the radiation pattern becomes asymmetric. We calculate the optimal distance between the two rods for maximum directivity in the z -direction. For this distance, we change the length of the reflector to obtain further enhancement of the radiated power in the positive z -direction. The same calculations are carried out after adding a slightly shorter element, the director, above the feed element. When excited by the dipole emitter, mutual coupling occurs between the single nanorods of the three-layer Yagi–Uda antenna. Because of the differences in length of the nanorods, the director (reflector) couples capacitively (inductively) to the feed element and the radiated power is directed into the positive z -direction (forward direction), whereas it is cancelled out in the negative z -direction (backward direction) [11] . Figure 2: Numerical directivity of the transmitting Yagi–Uda array coupled to dipole emitters. The polar plots show the numerically calculated directivity for ( a ) a single optical Yagi–Uda antenna, ( b ) a 2×2 array and ( c ) a 3×3 array. The calculated directivity of the xz plane is plotted in the left column and for the yz plane in the right column. Each antenna is fed by a dipole source (red spheres, 5 nm away from the feed element) with a dipole moment along the x -direction. The emitted wavelength of the dipole is 1500 nm. The black curves in the polar plots are the directivities of the corresponding emitter array without being coupled to optical antennas. Full size image The single dipole that is not coupled to a Yagi–Uda antenna shows the typical doughnut pattern with a maximal directivity of 1.5 (black curve). Adding the antenna, the directivity of the coupled system reaches 6 into the forward direction (red curve). In Figure 2b and c, the directivity patterns of the Yagi–Uda 2×2 array and 3×3 array (green and blue curve) and the patterns of the corresponding dipole arrays (black curves) are plotted. By adding more elements to the array ( Fig. 2a–c ), the directivity of the optical antenna array reaches higher peak directivities in the forward direction and the radiation beam becomes narrower. Clearly, an array of Yagi–Uda antennas directs the emission of dipole emitters more efficiently into the forward direction than a single antenna or just an array of dipoles. These directivities are obtained by coupling the antenna structures to dipole emitters that oscillate in phase. Using coherent nonlinear excitation and emission processes, such a phase-coherent feeding of the antennas in the array could be enabled. The numerical calculations take into account the near-field effects of the antennas on each other. For that reason the directivity does not reach the values one would obtain if the radiation pattern was calculated by pattern multiplication of the single-element pattern and the array factor [14] . Optical properties of the antenna array Because of reciprocity, the emitted radiation pattern of an antenna is equal to its receiving pattern. Experimentally, in the radiofrequency regime, it is common to determine the directive properties by measuring the load current of an antenna receiving radiation from a far away source. In the optical wavelength region, measurements of the near-field intensity by using aperturless Scanning Near-field Optical Microscopy as an indirect measurement of the current have been used to determine the reception patterns of linear antennas [22] . With our Yagi–Uda antenna being embedded into a dielectric matrix, we do not have access to the near-field region of the individual antenna elements. As an indirect measurement of the currents inside our antenna structure, we use ohmic losses. With the loss in power being proportional to the square of the current, we obtain the total loss in the antenna array P tot : with n being the number of antennas, I dir ( I feed , I ref ) being the current inside the director (feed element, reflector) and R being the resistance of the nanorod. As the antenna element length varies only by ∼ 10%, we can approximate their resistance to be equal. Equation (2) shows that we expect a higher ohmic loss if the induced currents are higher and not equally distributed over the elements. 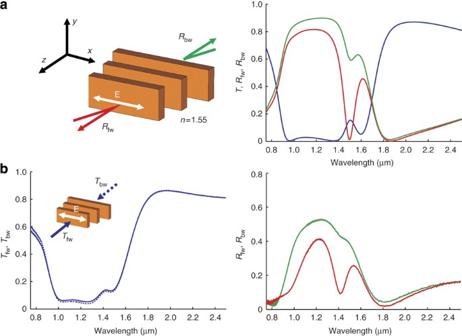Figure 3: Simulated spectra and experimental measurement of the optical Yagi–Uda array. (a) Numerical transmission and reflection spectra for forward and backward incidence on the antenna array as defined in the structure on the left. The white arrow indicates the polarization of the electric field vector along the axis of the rods. The blue curve shows the transmission spectrum, which is equal for both incidences. The red curve is the reflection spectrum for forward incidence and the green curve shows the reflection for backward incidence. (b) Experimental transmission (left) and reflection spectra (right) for forward incidence and backward incidence (right). The measured transmission is equal for both incidences, whereas the reflection spectra are different for forward and backward incidence. In Figure 3 , we investigate the optical properties in transmission and reflection of the array. In our experimental setup, the array receives radiation from two opposite directions. As depicted in Figure 3a, we define the forward direction for incident light from the director side and the backward direction for incident light from the reflector side. The light is polarized along the axis of the nanorods. The spectra in Figure 3a show the calculated transmission and reflection of the Yagi–Uda antenna array. By reciprocity, the transmitted intensity from the forward direction is equal to the transmitted intensity from the backward direction (blue curve), whereas more light incident from the backward direction is reflected (green curve) than from the forward direction (red curve). A significant difference between the two reflection spectra occurs at 1.5 μm, at which the radiation pattern shows the highest asymmetry. Nearly no light incoming from the positive z -direction is reflected at this wavelength. This is due to the resonant behaviour of the single Yagi–Uda nanoantenna, which has been designed to have maximum directivity into the forward direction at this wavelength. The experimental results are plotted in Figure 3b . The solid blue curve in the left plot shows the transmission spectrum for forward incidence, and the dashed blue curve for backward incidence. Three resonances occur, which are red- and blue-shifted compared with the particle plasmon resonance of equivalent single nanorod arrays ( Supplementary Fig. S1 ). Hence, the three layers couple to each other. As in the simulated spectra, the transmitted intensity is equal from both directions. In reflection (right plot in Fig. 3b ), more light is reflected for backward incidence than for forward incidence, which clearly confirms the broken forward–backward symmetry of directivity. By changing the polarization along the y -direction perpendicular to the long axes of the rods, the structural symmetry is not broken along the z -direction and no pronounced differences in the reflection spectra for forward and backward directions occur ( Supplementary Fig. S2 ). A significant dip in the reflection spectrum from forward direction occurs at λ =1.42 μm. We attribute the deviation of the resonance position to geometrical differences in the simulated and the fabricated structure. As the spacer layer is spin coated, the distance between the layers may slightly vary from the nominal 100 nm. Figure 3: Simulated spectra and experimental measurement of the optical Yagi–Uda array. (a ) Numerical transmission and reflection spectra for forward and backward incidence on the antenna array as defined in the structure on the left. The white arrow indicates the polarization of the electric field vector along the axis of the rods. The blue curve shows the transmission spectrum, which is equal for both incidences. The red curve is the reflection spectrum for forward incidence and the green curve shows the reflection for backward incidence. ( b ) Experimental transmission (left) and reflection spectra (right) for forward incidence and backward incidence (right). The measured transmission is equal for both incidences, whereas the reflection spectra are different for forward and backward incidence. Full size image Directive absorption of light by the antenna array The reflected intensity of the antenna array depends on the angle of incidence of the far-field radiation. As the transmission is equal for forward and backward incidence, the absorbed energy by the array is a function of the incident angle ( Supplementary Figs S3 and S4 ). 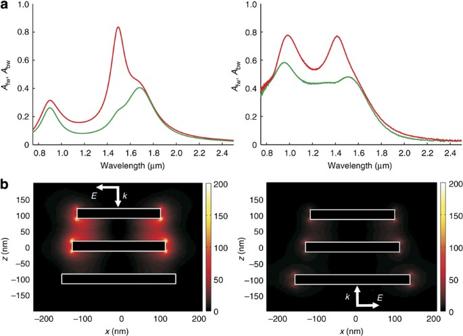Figure 4: Absorption of the incoming energy by the antenna array. (a) Absorption spectra deduced from simulated (left plot) and measured (right plot) spectra (A=1-T-R). At the resonance frequency the absorption shows the highest asymmetry for forward (red curves) and backward incidence (green curves). (b) Numerically calculated near-field intensity enhancement for forward (left plot) and backward incidence (right plot). The intensity at the tips of the feed element is significantly higher for forward incidence. Figure 4a compares the absorption spectra for the two opposite directions of incidence deduced from the simulated and the measured transmission and reflection spectra, following the relation A =1-T-R. At the resonance wavelength the absorption is maximally enhanced. Most of the energy is dissipated in the structure if the antenna array is excited from the + z -direction. This is confirmed by calculating the spectra with setting the imaginary part of the dielectric function, which is proportional to the specific ohmic resistance of the antenna material, to zero. In that case the reflection coefficients are equal for both incidence directions ( Supplementary Figs S5 and S6 ). In accordance with Equation (2), the significant difference in absorption at the resonant wavelength between forward and backward illumination is a clear indication that on forward illumination the induced currents are higher and distributed unevenly between the antenna elements. From the analogy with radiowave and microwave Yagi–Uda arrays, we suspect the currents to be concentrated in the feed elements. To verify our assumption, we extract the near-field intensities from our simulations. Figure 4b shows the near-fields for plane-wave illumination at the resonance wavelength ( λ =1.5 μm) from the forward direction (left plot) and the backward direction (right plot). For incidence from the forward direction, the electric near-field intensity is strongly enhanced at the feed element. For backward incidence these hot spots do not occur, which clearly confirms that the currents are distributed among the elements. In addition, the overall near-field for backward incident light is lower than that for forward incident light. This theoretical observation of the asymmetric near-field intensities matches very well with our observations in near-field experiments of planar Yagi–Uda antennas ( Supplementary Figs S7 and S8 ). There, we find that the near-field intensity is either distributed over several elements for backward illumination ( Supplementary Fig. S8, right) or concentrated on the feed element for forward incidence ( Supplementary Fig. S8, left). Figure 4: Absorption of the incoming energy by the antenna array. ( a ) Absorption spectra deduced from simulated (left plot) and measured (right plot) spectra ( A =1-T-R). At the resonance frequency the absorption shows the highest asymmetry for forward (red curves) and backward incidence (green curves). ( b ) Numerically calculated near-field intensity enhancement for forward (left plot) and backward incidence (right plot). The intensity at the tips of the feed element is significantly higher for forward incidence. Full size image In a phased array, each element is driven independently with a defined phase and amplitude. The angular pattern depends on the phase shift between the elements. The concept has been applied for antenna structures in the far infrared, using an array of λ/2 dipole antennas [23] . We propose to use the optical 3D Yagi–Uda antenna array for beam steering applications in the optical regime at λ =1500 nm. Because of the high directivity of the array, light can be efficiently directed out of the substrate into a well-defined direction. 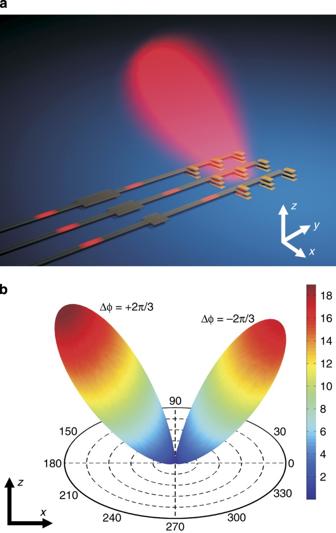Figure 5: Phased array of optical Yagi–Uda antennas. (a) Schematic representation of a 3×3 Yagi–Uda antenna array that is fed by a phase modulating feeding circuit through plasmonic waveguides. A phase difference of the incoming light signal is induced by phase shifters. The direction of the emitted light cone depends on the phase difference between adjacent antennas. (b) Numerical three-dimensional directivity plots of the 3×3 phased array. The beam is scanned in thexzplane from approximately −30° to +30°. This is obtained by inducing a phase shift of Δφ=+2π/3 and Δφ=−2π/3 in thex-direction. The radiation patterns show different peak directivities as the antennas are fed at one end of the feed elements. Figure 5a depicts a schematic view of a 3×3 Yagi–Uda antenna array in which the feed elements are connected to plasmonic waveguides [24] or high-index dielectric waveguides to avoid major losses in the waveguides [25] . Each Yagi–Uda antenna is addressed independently and the phase of the feeding circuit is controlled by phase modulators. Inducing a phase shift in the x -direction between adjacent Yagi–Uda antennas of +2π/3 and −2π/3, leads to a beam steering in the xz plane from approximately −30° to +30°, as it is calculated in Figure 5b . The slight asymmetry in the values of the peak directivity of the two patterns occurs as the antennas are fed by the waveguides to the left side of the feed elements as it is shown in Figure 5a . Figure 5: Phased array of optical Yagi–Uda antennas. (a ) Schematic representation of a 3×3 Yagi–Uda antenna array that is fed by a phase modulating feeding circuit through plasmonic waveguides. A phase difference of the incoming light signal is induced by phase shifters. The direction of the emitted light cone depends on the phase difference between adjacent antennas. ( b ) Numerical three-dimensional directivity plots of the 3×3 phased array. The beam is scanned in the xz plane from approximately −30° to +30°. This is obtained by inducing a phase shift of Δφ=+2π/3 and Δφ=−2π/3 in the x -direction. The radiation patterns show different peak directivities as the antennas are fed at one end of the feed elements. Full size image In conclusion, we have demonstrated experimentally that the amount of electromagnetic energy dissipated by our Yagi–Uda array highly depends on the angle of incidence. It becomes maximal for forward incident light, in which most of the energy is absorbed by the feed elements. This may open a new pathway to highly sensitive detection of infrared radiation by combining the antenna array with a suitable focal-plane array. In the future, the 3D geometry provides a possible extension to an optical phased array, which is a completely new perspective for controlling light on the nanoscale by enabling narrow-angle beam steering. Moreover, optical nanoantenna point-to-point connections with switching functionalities could become reality. Structure fabrication For the fabrication, a Raith e_LiNE electron beam lithography (EBL) system is used. The acceleration voltage is set to 20 kV. We use a Infrasil 302 quartz glass as a substrate. A double-layer PMMA is spin coated onto the substrate and the solvent is evaporated by baking the sample for 5 min at 160 °C after each resist layer. After structuring the resist with the EBL system and subsequent developing of the sample, a 3-nm adhesion layer of chromium and 30 nm of gold are evaporated. A standard lift-off procedure removes the remaining resist. The polymer PC403 serves as a dielectric spacer and smoothens the substrate surface for the consecutive layer. The process is repeated for each layer in which the coordinate system in the EBL is defined by fixed gold markers on the substrate for each layer. Structure characterization The electron micrographs of the fabricated structures are taken with a Hitachi S-4800 scanning electron microscope. Figure 1b shows a tilted view of the array structure in which the acceleration voltage is set to 15 kV. Optical far-field measurements Transmittance and reflectance spectra of the antenna array are obtained using a Fourier-transform infrared spectrometer (Bruker Vertex 80, tungsten lamp) combined with an infrared microscope (Bruker Hyperion) equipped with a ×15 Cassegrain objective (numerical aperture, NA=0.4), a liquid N 2 -cooled MCT 77K detector and a Si diode detector. The polarization of the incident light is controlled by an infrared polarizer. The measured spectra are normalized with respect to a bare glass substrate for transmittance and a gold mirror for reflectance. The forward and backward spectra are recorded by flipping the sample in the optical light path. Numerical simulations The numerical results are obtained by using the software package CST Microwave Studio, Darmstadt, Germany. The far-field pattern of Figure 2 is calculated with the antenna structure being embedded in a homogenous environment with a refractive index of n PC403 =1.55 to account for the dielectric matrix in which the fabricated structure is embedded. For the array configuration ( Fig. 2b and c ), each Yagi–Uda antenna is implemented into the calculation domain and each antenna is fed independently by an electric dipole source. The dipole moment of the source is aligned with the long axis of the feed element and placed 5 nm away. Periodic boundaries are set for the transmittance and reflectance spectra in Figure 3a and the near-field distributions of Figure 4b . As optical parameters, we use the refractive index of PC403, n PC403 =1.55 and the quartz substrate refractive index, n glass =1.46. In all simulations the permittivity of gold in the near-infrared spectral regime is described by a Drude model fitted to experimental data [26] with plasma frequency ω pl =1.37×10 16 rad s −1 and damping constant γ =1.2×10 14 rad s −1 . How to cite this article: Dregely, D. et al . 3D optical Yagi–Uda nanoantenna array. Nat. Commun. 2:267 doi: 10.1038/ncomms1268 (2011).